Helium penetrates into silica glass and reduces its compressibility SiO 2 glass has a network structure with a significant amount of interstitial voids. Gas solubilities in silicates are expected to become small under high pressure due to compaction of voids. Here we show anomalous behaviour of SiO 2 glass in helium. Volume measurements clarify that SiO 2 glass is much less compressible than normal when compressed in helium, and the volume in helium at 10 GPa is close to the normal volume at 2 GPa. X-ray diffraction and Raman scattering measurements suggest that voids are prevented from contracting when compressed in helium because helium penetrates into them. The estimated helium solubility is very high and is between 1.0 and 2.3 mol per mole of SiO 2 glass at 10 GPa, which shows marked contrast with previous models. These results may have implications for discussions of the Earth's evolution as well as interpretations of various high-pressure experiments, and also lead to the creation of new materials. SiO 2 glass is an archetypal network-forming glass [1] , [2] , [3] and widely used as a high-performance material. SiO 2 glass is compressible among silicates (or oxides) [4] , [5] , [6] , [7] because it has a structure with a significant amount of interstitial voids [8] . Elastic softening and permanent densification of SiO 2 glass under high pressure are interesting issues in physics and materials science [4] , [5] , [6] , [9] , [10] , [11] , [12] and closely related to deformation and compaction of these voids. Information on the pressure dependence of its structure and density is also important in geophysics, because glasses can be considered as the analogue material of melts [11] , [13] . Helium is monatomic and the smallest molecule, and therefore is used as a light inert gas. It is also widely used as the most ideal pressure medium in high-pressure experiments, because it remains soft enough to hold samples under nearly hydrostatic conditions over a wide pressure range [14] . The isotopic ratio of helium is useful as a tracer of the Earth's evolution [15] , [16] , [17] , [18] . It seems likely that helium atoms dissolve in the voids in SiO 2 glass, considering that SiO 2 glass has a structure with a significant amount of interstitial voids and helium is the smallest molecule. In fact, the maximum solubility of helium in SiO 2 glass has been estimated to be as much as 0.1 mol per mole of SiO 2 glass, based on measurements up to about 0.1 GPa and a statistical thermodynamical model [19] . On the other hand, gas solubilities are expected to decrease drastically at high pressures due to compaction of voids [16] , [18] . However, these well-accepted models cannot explain the experimental data shown below. In this article, we show anomalous behaviour of SiO 2 glass in helium under high pressure. It was found that SiO 2 glass is much less compressible than normal when compressed in a helium medium, suggesting that the voids in SiO 2 glass are prevented from contracting, because a large amount of helium penetrates into these voids. These results may impact discussions of the Earth's evolution as well as interpretations of various high-pressure experiments, and, potentially, also lead to the creation of new materials. Pressure dependence of the volume of SiO 2 glass in helium The volume change ( V / V 0 ) was determined by measuring the change in the size of the bulk sample in optical-microscope images [5] , [20] . 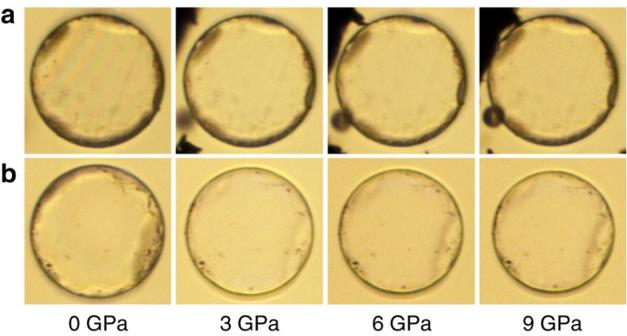Figure 1: Pressure dependence of the sample size of SiO2glass in a diamond-anvil cell. Typical photographs of SiO2glass in a helium medium (rigid) are shown in (a) and those in a methanol-ethanol medium (normal) are shown in (b). The photograph at 0 GPa in (a) was taken without helium. In (a) at 3, 6, and 9 GPa, a ruby ball and a fraction of deformed gasket are seen. An initial diameter of the sample was about 80 μm in both (a) and (b). Although the samples are almost the same size at 0 GPa, the sample in methanol-ethanol is obviously smaller than that in helium at 9 GPa. Typical images are shown in Figure 1 . 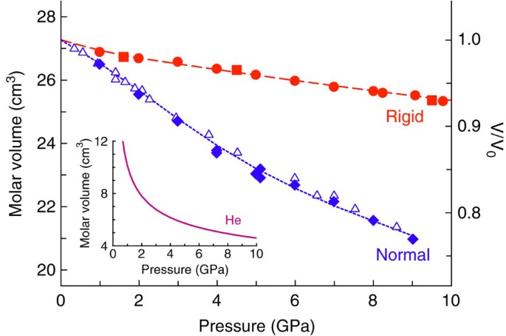Figure 2: Pressure dependence of the volume of SiO2glass. The volume change of SiO2glass in a helium medium (rigid) is much smaller than that in a methanol-ethanol medium (normal). The red filled circles and squares represent our data in two independent runs in helium. The red broken line is a guide for the eyes. The blue filled diamonds represent our data in methanol-ethanol. The blue open triangles and the blue dotted line represent the data in methanol-ethanol by Meade & Jeanloz5and Tsioket al.6, respectively. The volume change in methanol-ethanol measured in this study is consistent with those in previous studies, indicating that the low compressibility in helium cannot be attributed to problems in the sample and/or method of measurements. The pressure dependence of the volume of helium is also shown for comparison in the inset28,29,30. The pressure dependence of the volume of SiO 2 glass is shown in Figure 2 . As seen in Figures 1 and 2 , the volume change of SiO 2 glass in a helium medium is much smaller than that in a mixture of methanol-ethanol medium. The volume in helium at 10 GPa is close to that in methanol-ethanol at 2 GPa. At pressures below 20 GPa, SiO 2 glass has a network structure consisting of SiO 4 tetrahedra. The SiO 4 tetrahedra are very incompressible [21] , [22] , [23] , and the high compressibility of SiO 2 glass is ascribed to changes in the intermediate-range order, that is, compaction of voids [12] . Therefore, this low compressibility of SiO 2 glass in helium is considered to be caused by occupation of voids by helium atoms. Figure 1: Pressure dependence of the sample size of SiO 2 glass in a diamond-anvil cell. Typical photographs of SiO 2 glass in a helium medium (rigid) are shown in ( a ) and those in a methanol-ethanol medium (normal) are shown in ( b ). The photograph at 0 GPa in ( a ) was taken without helium. In ( a ) at 3, 6, and 9 GPa, a ruby ball and a fraction of deformed gasket are seen. An initial diameter of the sample was about 80 μm in both ( a ) and ( b ). Although the samples are almost the same size at 0 GPa, the sample in methanol-ethanol is obviously smaller than that in helium at 9 GPa. Full size image Figure 2: Pressure dependence of the volume of SiO 2 glass. The volume change of SiO 2 glass in a helium medium (rigid) is much smaller than that in a methanol-ethanol medium (normal). The red filled circles and squares represent our data in two independent runs in helium. The red broken line is a guide for the eyes. The blue filled diamonds represent our data in methanol-ethanol. The blue open triangles and the blue dotted line represent the data in methanol-ethanol by Meade & Jeanloz [5] and Tsiok et al . [6] , respectively. The volume change in methanol-ethanol measured in this study is consistent with those in previous studies, indicating that the low compressibility in helium cannot be attributed to problems in the sample and/or method of measurements. The pressure dependence of the volume of helium is also shown for comparison in the inset [28] , [29] , [30] . 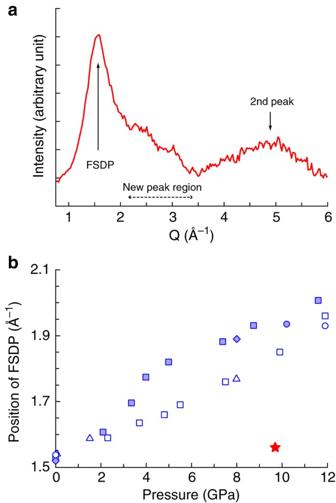Figure 3: X-ray diffraction pattern and the FSDP position of SiO2glass in helium. (a) The X-ray diffraction pattern of SiO2glass in helium measured at 10 GPa. The FSDP is considered to be associated with the periodicity of ordering of the rings consisting of SiO4tetrahedra2,3. A new peak at around 3 Å−1, which is considered to be associated with the periodicity of chemical ordering of Si-O pairs3, appears above 3–4 GPa in the normal case12,22. An indication of this new peak is observed between 2.2 and 3.4 Å−1. No major changes in the second peak at around 5 Å−1is observed as normal. (b) Pressure dependence of the position of the FSDP of SiO2glass. The FSDP position in helium (red star) is significantly different from those in previous studies. The blue open symbols represent the FSDP position at room temperature (squares: Inamuraet al.12, circles: Funamori & Sato37, triangles: Benmoreet al.22). The blue filled symbols represent the FSDP position at high temperatures or under conditions where the structure and/or deviatoric stresses have been relaxed (diamonds: Meadeet al.21, squares: Inamuraet al.12, circles: Sato & Funamori23). As helium is in a liquid state at 10 GPa, the FSDP position was not affected by deviatoric stresses. Full size image X-ray diffraction pattern of SiO 2 glass in helium The X-ray diffraction pattern of SiO 2 glass in a helium medium obtained at 10 GPa and the pressure dependence of the position of the first sharp diffraction peak (FSDP) of SiO 2 glass are shown in Figure 3a,b , respectively. As seen in Figure 3b , the position of the FSDP in helium is significantly different from those in previous studies. The FSDP is associated with the presence of the intermediate-range order and considered to arise from the periodicity of ordering of the rings consisting of SiO 4 tetrahedra [2] , [3] . The position of the FSDP in helium at 10 GPa is close to that in previous studies at 1–2 GPa. This result is consistent with the fact that the volume in helium at 10 GPa is close to that in methanol-ethanol at 2 GPa. An indication of a peak is observed at around 2.2–3.4 Å −1 . In this region, no peak is observed at ambient pressure, and a new peak appears at high pressures. However, the new peak has not been observed so far at about 2 GPa [12] , [22] , suggesting that the structure of SiO 2 glass in helium at 10 GPa is not identical to the normal structure at 1–2 GPa. Figure 3: X-ray diffraction pattern and the FSDP position of SiO 2 glass in helium. ( a ) The X-ray diffraction pattern of SiO 2 glass in helium measured at 10 GPa. The FSDP is considered to be associated with the periodicity of ordering of the rings consisting of SiO 4 tetrahedra [2] , [3] . A new peak at around 3 Å −1 , which is considered to be associated with the periodicity of chemical ordering of Si-O pairs [3] , appears above 3–4 GPa in the normal case [12] , [22] . An indication of this new peak is observed between 2.2 and 3.4 Å −1 . No major changes in the second peak at around 5 Å −1 is observed as normal. ( b ) Pressure dependence of the position of the FSDP of SiO 2 glass. The FSDP position in helium (red star) is significantly different from those in previous studies. The blue open symbols represent the FSDP position at room temperature (squares: Inamura et al . [12] , circles: Funamori & Sato [37] , triangles: Benmore et al . [22] ). The blue filled symbols represent the FSDP position at high temperatures or under conditions where the structure and/or deviatoric stresses have been relaxed (diamonds: Meade et al . [21] , squares: Inamura et al . [12] , circles: Sato & Funamori [23] ). As helium is in a liquid state at 10 GPa, the FSDP position was not affected by deviatoric stresses. 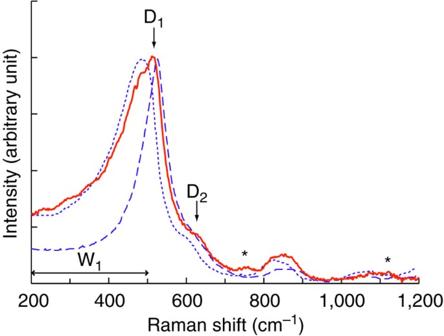Figure 4: Raman spectrum of SiO2glass in helium. The spectrum in helium measured at 10 GPa (red line) is shown together with the spectra in argon at 3.6 and 8.0 GPa (blue dotted and broken lines, respectively: Hemleyet al.10) for comparison. The peaks with an asterisk may be due to the fluorescence of diamond anvils. TheW1band at 200–500 cm−1is considered to be associated with Si-O-Si bending motion24. Because SiO2glass mainly consists of six-membered rings at ambient pressure, theW1band is considered to mainly reflect the behaviour of six-membered rings. The feature of theW1band in helium at 10 GPa is similar to that in the normal spectrum (that is, in argon) at 3.6 GPa. TheD1andD2defect bands at around 500 and 650 cm−1are considered to be associated with the breathing modes of four- and three-membered rings, respectively25. The position of theD1band is between those in the normal spectra at 3.6 and 8.0 GPa, and the position of theD2band is similar to that in the normal spectrum at 8.0 GPa. It is suggested that large voids are less compressible than normal and small voids are as compressible as normal. Full size image Raman spectrum of SiO 2 glass in helium The Raman spectrum of SiO 2 glass in a helium medium obtained at 10 GPa is shown in Figure 4 . It has been reported that a characteristic Raman band at around 500 cm −1 continuously shifts to higher frequencies and becomes sharp with increasing pressure [10] . However, the spectrum in helium at 10 GPa is significantly different from those reported in previous studies. This spectrum seems to be a mixture of the normal spectra obtained at 3.6 and 8.0 GPa. The diffuse band at 200–500 cm −1 , denoted as W 1 , is considered to be mainly associated with vibrational motions of six-membered rings [10] , [24] . On the other hand, two sharp bands at around 500 and 650 cm −1 , denoted as D 1 and D 2 , are the defect bands and assigned to the breathing modes of four- and three-membered rings, respectively [25] . In the spectrum in helium at 10 GPa, the feature of the W 1 band is similar to that in the normal spectrum at 3.6 GPa, the position of the D 1 band is intermediate between those in the normal spectra at 3.6 and 8.0 GPa, and the position of the D 2 band is similar to that in the normal spectrum at 8.0 GPa. Void size is closely related to ring configurations [26] , and therefore these observations suggest the following picture. Voids inside large rings, such as six-membered rings, are much less compressible than normal, because these voids are preferentially occupied by helium atoms. Voids inside medium rings, such as four-membered rings, are less compressible than normal, because these voids are partly occupied by helium atoms. Voids inside small rings, such as three-membered rings, are as compressible as normal, because these voids are too small to be occupied by helium atoms. Figure 4: Raman spectrum of SiO 2 glass in helium. The spectrum in helium measured at 10 GPa (red line) is shown together with the spectra in argon at 3.6 and 8.0 GPa (blue dotted and broken lines, respectively: Hemley et al . [10] ) for comparison. The peaks with an asterisk may be due to the fluorescence of diamond anvils. The W 1 band at 200–500 cm −1 is considered to be associated with Si-O-Si bending motion [24] . Because SiO 2 glass mainly consists of six-membered rings at ambient pressure, the W 1 band is considered to mainly reflect the behaviour of six-membered rings. The feature of the W 1 band in helium at 10 GPa is similar to that in the normal spectrum (that is, in argon) at 3.6 GPa. The D 1 and D 2 defect bands at around 500 and 650 cm −1 are considered to be associated with the breathing modes of four- and three-membered rings, respectively [25] . The position of the D 1 band is between those in the normal spectra at 3.6 and 8.0 GPa, and the position of the D 2 band is similar to that in the normal spectrum at 8.0 GPa. It is suggested that large voids are less compressible than normal and small voids are as compressible as normal. Full size image Estimation of helium solubility in SiO 2 glass A model on the distribution of the size of interstitial void sites in SiO 2 glass has been proposed based on its similarity to cristobalite in interstitial structure [8] , [26] , [27] . According to this model, the distribution of void size is log-normal, and the total number of void sites is 2.22×10 22 cm −3 , that is, 1.00 mol per mole of SiO 2 glass. As described earlier, the maximum helium solubility was previously estimated to be 0.1 mol per mole of SiO 2 glass [19] . This value has been ascribed to the maximum number of void sites available to helium, which has a radius of 1.3 Å (ref. 8 ). However, as described below, this model cannot explain the solubility under high pressure. 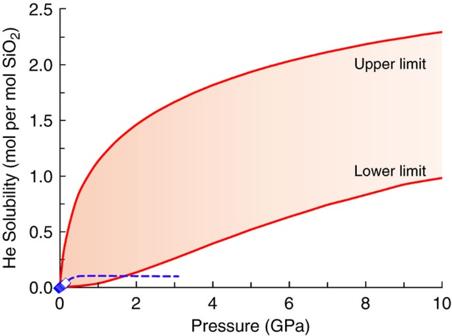Figure 5: Helium solubility in SiO2glass. Lower and upper limits on helium solubility in SiO2glassCHeare estimated from the volumes with the inequalities,VSiO2G(rigid)−VSiO2G(normal)<CHeVHe<VSiO2G(rigid)−VSiO2G(sixfold).VSiO2G(rigid),VSiO2G(normal), andVHeare shown inFigure 2.VSiO2G(sixfold) is calculated by using a third-order Birch-Murnaghan equation of state with the zero-pressure volume, bulk modulus, and its pressure derivative of 15.5 cm3/mol, 190 GPa, and 4.5, respectively7. Helium solubility reported in a low-pressure range up to 0.1 GPa is shown for comparison (blue open diamonds: Shelby19). An extrapolation of the low-pressure data based on a statistical thermodynamical model (blue broken line: Shelby19) cannot explain the volume changes measured at higher pressures. The helium solubility in SiO 2 glass is estimated from the volumes of SiO 2 glass and helium as shown in Figure 5 . A lower limit on helium solubility in SiO 2 glass is estimated as follows. At a given pressure and temperature, materials behave so as to minimize the Gibbs free energy G = U + PV − TS . As the PV term is dominant under high pressure, it is assumed that the inequality, V SiO2G (rigid)< C He V He + V SiO2G (normal), holds in the first approximation. Here V SiO2G (rigid) and V SiO2G (normal) represent the molar volume of SiO 2 glass in helium and that under normal conditions, respectively, and C He and V He represent helium solubility in SiO 2 glass and the molar volume of helium, respectively. As shown in Figure 5 , a lower limit on helium solubility increases almost linearly with increasing pressure and reaches 1.0 mol per mole of SiO 2 glass at 10 GPa. Figure 5: Helium solubility in SiO 2 glass. Lower and upper limits on helium solubility in SiO 2 glass C He are estimated from the volumes with the inequalities, V SiO2G (rigid)− V SiO2G (normal)< C He V He < V SiO2G (rigid)− V SiO2G (sixfold). V SiO2G (rigid), V SiO2G (normal), and V He are shown in Figure 2 . V SiO2G (sixfold) is calculated by using a third-order Birch-Murnaghan equation of state with the zero-pressure volume, bulk modulus, and its pressure derivative of 15.5 cm 3 /mol, 190 GPa, and 4.5, respectively [7] . Helium solubility reported in a low-pressure range up to 0.1 GPa is shown for comparison (blue open diamonds: Shelby [19] ). An extrapolation of the low-pressure data based on a statistical thermodynamical model (blue broken line: Shelby [19] ) cannot explain the volume changes measured at higher pressures. Full size image The solubility of more than 1.0 mol per mole of SiO 2 glass at 10 GPa cannot be explained by the conventional model on void-size distribution [8] . The radius of helium at 10 GPa is calculated to be 1.1 Å, assuming that a helium atom is a hard sphere and in a close-packed configuration under high pressure [28] , [29] , [30] . Only less than half of all void sites are available with this radius. It is also difficult to assume that large void sites are occupied by two or more helium atoms, because the maximum diameter of void sites is about 4 Å in this model. Moreover, the fact that the difference between V SiO2G (rigid) and V SiO2G (normal) continuously increases with increasing pressure up to 10 GPa is not consistent with the model in which gas solubilities decrease drastically at high pressures due to compaction of voids [16] , [18] . It may be appropriate to consider that helium atoms are continuously stacked in three-dimensionally connected voids, because voids in SiO 2 glass may not be isolated [8] . A total effective volume of voids, which can be occupied by helium atoms, is roughly estimated as follows. It is assumed that the voids effectively and completely collapse when SiO 2 glass transforms to a high-pressure sixfold-coordinated form, that is, a structure consisting of SiO 6 octahedra. Under this assumption, a total effective volume of voids in fourfold-coordinated SiO 2 glass is considered to be equal to the difference in volume between fourfold- and sixfold-coordinated SiO 2 glasses. Therefore, an upper limit on helium solubility in SiO 2 glass is estimated with the inequality, V SiO2G (rigid)− V SiO2G (sixfold)> C He V He . Here V SiO2G (sixfold) represents the molar volume of sixfold-coordinated SiO 2 glass, and is available in the literature [7] . As shown in Figure 5 , the helium solubility may be between 1.0 and 2.3 mol per mole of SiO 2 glass at 10 GPa. The data in the previous study at around 0.1 GPa [19] fall within our estimation, although the extrapolation of this data is not consistent with our estimation. Our findings motivate us to reconsider various conventional discussions. As described earlier, helium is considered to be the most ideal pressure medium that holds samples under nearly hydrostatic conditions at high pressures [14] . However, it should be used with caution. In fact, it is well known that gas atoms penetrate into microporous crystals (that is, crystals having larger voids with a diameter up to 20 Å), such as fullerenes [31] , zeolites [32] , and clathrates [33] , and affect their compression behaviour. Our results suggest the possibility that helium may cause (or may have caused) some problems also in experiments on ordinary materials with voids. From a geophysical viewpoint, the fact that helium solubility in SiO 2 glass at high pressures is completely different from the estimation based on the data at low pressures [19] may suggest the necessity of reconsidering conventional models on degassing from the mantle and other relevant events in the Earth's history. The interaction between SiO 2 glass and other noble gases with larger atomic radii may be similar to the case for helium qualitatively, although it must be much smaller quantitatively. Therefore, recent experiments on the dissolution of noble gases in silicates under high pressure should be carefully interpreted. In many of these experiments, gas solubilities have been estimated by heating crystals to be melted in noble gas mediums and measuring the amount of gas contained in recovered glasses [16] , [18] . Our results suggest that the existence of a large amount of gas may affect the behaviour of voids in silicates, and therefore the behaviour of noble gases in silicates may change with their partial pressure, which is much higher in experiments than in the Earth. In addition, these glasses may have already been degassed when recovered to ambient conditions. Finally, our findings may open up a novel approach to synthesizing new materials. When helium atoms occupy voids in materials at high pressures, these materials are compressed not only from the outside but also from the inside. This is very different from normal compression. Therefore, new phases may be synthesized at high pressures and/or recovered to ambient pressure. For example, cristobalite is highly likely to transform to a new structure, because it has a structure similar to SiO 2 glass [1] , [8] , [26] , [27] . On the basis of this assumption, we have recently compressed cristobalite in a helium medium and observed a new phase at 10 GPa, which shows diffraction peaks at larger d values. Quartz has a denser structure than cristobalite, but it has been reported to have been recovered in a new metastable crystalline phase by compression in helium [34] . This might be related to dissolution of helium in voids. It is also possible that other small gas molecules, such as H 2 , might dissolve in voids. Various combinations of materials with voids and small molecules will be studied in the future. Some polymers have a structure with very large voids [35] , and are able to accommodate relatively large gas molecules, such as CH 4 and CO 2 . These large voids generally contract at low pressures of a few thousand atmospheres. It may be possible to create new useful materials with compression in gases. Sample preparation SiO 2 glass with 99.99% purity in the form of a wire having a diameter of 80 μm was prepared by FHP Engineering Limited and used as the sample. The X-ray diffraction pattern and Raman spectrum of this sample agreed with those reported in previous studies [3] , [10] , [12] , [21] , [22] , [24] , [25] , [36] , [37] at ambient conditions. It was cut and polished to a thickness of about 50 μm and then put in a rhenium gasket for diamond-anvil experiments. Diamond-anvil experiments High-pressure experiments were conducted with a diamond-anvil cell at room temperature. Anvils having a 600 μm flat culet were used. Pressure was determined by the ruby-fluorescence method with the quasihydrostatic scale [38] . Three independent runs were conducted, with a helium pressure medium in runs 1 and 2, and with a 4:1 mixture of methanol-ethanol medium in run 3 for comparison. The culet of the anvil and the surface of the sample were not able to be focused simultaneously by an optical microscope throughout the experiments. This ensured that the samples did not bridge between the anvils and were not affected by deviatoric stresses. The volume change ( V / V 0 ) of the sample was measured in all the runs. X-ray diffraction and Raman scattering measurements were carried out in run 1 at the highest pressure (that is, 10 GPa). V / V 0 was determined by measuring the change in the size of the sample in optical-microscope images [5] , [20] ( Fig. 1 ). Glasses can be assumed to be isotropically compressed (whereas crystals are not isotropically compressed, and therefore the volume change of crystals is generally determined by an X-ray diffraction method). X-ray diffraction measurements were carried out by using an angle-dispersive method with 25 keV monochromatic X-rays and an imaging plate detector at BL-18C of Photon Factory. The exposure time was 10 and 5 h for the sample and background, respectively. Raman scattering measurements were carried out by using the 488 nm line of an argon ion laser for excitation in a 150° light-scattering geometry and a ×10 micro-optical spectrometer system consisting of a longpass filter, an imaging spectrometer, and a Peltier-cooled charge-coupled device. The spectrum was corrected by measuring the background. How to cite this article: Sato, T. et al . Helium penetrates into silica glass and reduces its compressibility. Nat. Commun. 2:345 doi: 10.1038/ncomms1343 (2011).